Deciphering the importance of the palindromic architecture of the immunoglobulin heavy-chain 3’ regulatory region The IgH 3’ regulatory region ( 3’RR ) controls class switch recombination (CSR) and somatic hypermutation (SHM) in B cells. The mouse 3’RR contains four enhancer elements with hs1,2 flanked by inverted repeated sequences and the centre of a 25-kb palindrome bounded by two hs3 enhancer inverted copies ( hs3a and hs3b ). hs4 lies downstream of the palindrome. In mammals, evolution maintained this unique palindromic arrangement, suggesting that it is functionally significant. Here we report that deconstructing the palindromic IgH 3’RR strongly affects its function even when enhancers are preserved. CSR and IgH transcription appear to be poorly dependent on the 3’RR architecture and it is more or less preserved, provided 3’RR enhancers are present. By contrast, a ‘palindromic effect’ significantly lowers V H germline transcription, AID recruitment and SHM. In conclusion, this work indicates that the IgH 3’RR does not simply pile up enhancer units but also optimally exposes them into a functional architecture of crucial importance. Lymphopoiesis is coupled with programmed accessibility of Ig genes to transcription and to several major transcription-dependent DNA-remodelling events [1] , [2] . Multiple cis -regulatory elements located 5’ and 3’ of constant ( C ) genes control B-cell ontogeny. Among 5’ elements, the intronic Eμ enhancer is reported as a master control element of V(D)J recombination [3] , [4] . The IgH 3’ regulatory region ( 3’RR ), which encompasses the four transcriptional enhancers hs3a, hs1,2 , hs3b and hs4 , controls μ-transcription in mature B cells [5] , and is the master element controlling conventional class switch recombination (CSR) [6] , [7] , locus suicide recombination [8] and somatic hypermutation (SHM) [9] but with little role in V(D)J recombination, except for silencing early transcription in pro-B cells [10] , [11] , [12] . The mouse 3’RR contains four enhancer elements ( hs3a , hs1,2 , hs3b and hs4 ) with hs1,2 flanked by inverted repeated intervening sequences ( IRIS ) and the centre of a >25-kb palindrome bounded by 2 inverted copies of the hs3 enhancers ( hs3a and hs3b ) refs 2 , 13 . hs4 lies downstream of the palindrome. The modest activity of each of the 3’RR elements in vitro , however, contributes to a synergic and potent global effect of the 3’RR in transgenes, especially when its ‘palindromic’ architecture is maintained [14] . In humans, each of the two 3’RR located downstream of Cα1 and Cα2 contains three enhancer elements similar to mouse hs3 , hs1,2 and hs4 , with hs1,2 being also flanked by IRIS . Beyond divergence of hs1,2 -flanking sequences, evolution maintained a ‘quasi-palindromic’ organisation in all mammals for which sequence is available, making it tempting to speculate that this unique arrangement is of significant importance for the regulatory region function [15] . To explore the role of the 3’RR palindromic architecture in the context of the endogenous locus, we analysed two newly generated transgenic mice: hs3a + IRIS + hs1,2 -deficient mice (called ΔleftPAL mice in this study) lacking the 11.5-kb left half of the 3’RR palindrome (deconstructing palindrome and deleting two enhancer elements) and Δ IRIS mice with the same left-half deletion of the palindrome but with reintroduction of a inverted hs3a and hs1,2 enhancers (deconstructing the palindrome by fully eliminating left-side IRIS while maintaining all four core enhancer elements). We report that the deconstruction of the IgH 3’ palindrome widely affects SHM but only marginally affects CSR, showing that the unique architecture of the IgH locus 3’ boundary crucially determines the full functional expression of the IgH 3’RR transcriptional enhancers. Generation of ΔleftPAL and ΔIRIS mice The location of the 3’RR on the IgH locus is reported in Fig. 1a . 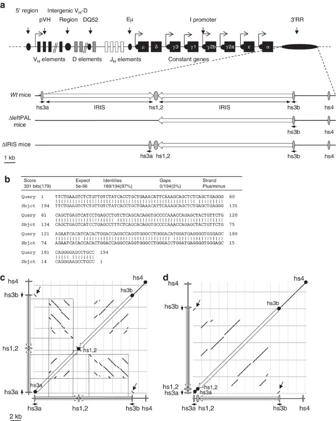Figure 1: Palindromic structure of theIgH 3’RR. (a) Upper part: The mouseIgHlocus (not on the scale). Lower part: The3’RRwith its four enhancer elements and theIRIS(on the scale). ΔleftPAF and ΔIRIS mice are represented. (b) Sequence and homology betweenhs3aandhs3benhancers (in opposite orientation in the chromosome). (c,d) DNA sequence dot-plot of the3’RRinwt(c) and ΔIRISmice (d) showing self similarity. The main diagonal represents the sequence alignment with itself. Parallel lines to the main diagonal represent repetitive patterns within the sequence (that is, tandem repeat), whereas perpendicular lines to the main diagonal represent similar but inverted sequences, thus allowing to identify the palindromic structures (dotted lines). The inversion ofhs3aenhancer (black arrows) and the deletion of the intervening sequences betweenhs3aandhs1,2in ΔIRISmice totally disrupts the palindromic structure, despite the presence of all enhancer elements. Figure 1b reports the 97% homology between hs3a and hs3b (in inverse orientation on the chromosome). Dot-plot analysis of the 3’RR DNA fragment encompassing hs3a to hs4 reveals locations of tandem repeats and inverted sequences defining the 3’RR palindromic structure ( Fig. 1c ). Inversion of hs3a and deletion of intervening sequences between hs3a and hs1,2 in Δ IRIS mice totally disrupt the palindromic structure, while maintaining the presence of all 3’RR enhancers. The ES14 cell line was used to generate ΔleftPAL and Δ IRIS mice. The gene-targeting vector replaced the 11.5-kb genomic fragment encompassing the IRIS and hs3a / hs1,2 enhancers with a floxed neo R cassette (ΔleftPAL mutation; Supplementary Fig. 1 ). Specific 5’ and 3’ PCR allowed the selection of 8 out of 984 clones. Another gene-targeting vector replaced the genomic fragment encompassing the IRIS and hs3a / hs1,2 enhancers with a cassette including an inverted copy of hs3a plus hs1,2 enhancer and a floxed neo R cassette (Δ IRIS mutation; Supplementary Fig. 1 ). Inserting hs3a in inverted orientation allowed us to completely suppress any dyad symmetry around hs1,2 without deleting any enhancer sequence ( Fig. 1c,d ). Specific 5’ and 3’ PCR allowed the selection of 6 out of 536 clones. After germline transmission, breeding with cre-expressing mice allowed the derivation of ΔleftPAL and Δ IRIS mice after cre-deletion of neo R ( Supplementary Fig. 1 ). Figure 1: Palindromic structure of the IgH 3’RR . ( a ) Upper part: The mouse IgH locus (not on the scale). Lower part: The 3’RR with its four enhancer elements and the IRIS (on the scale). ΔleftPAF and ΔIRIS mice are represented. ( b ) Sequence and homology between hs3a and hs3b enhancers (in opposite orientation in the chromosome). ( c , d ) DNA sequence dot-plot of the 3’RR in wt ( c ) and Δ IRIS mice ( d ) showing self similarity. The main diagonal represents the sequence alignment with itself. Parallel lines to the main diagonal represent repetitive patterns within the sequence (that is, tandem repeat), whereas perpendicular lines to the main diagonal represent similar but inverted sequences, thus allowing to identify the palindromic structures (dotted lines). The inversion of hs3a enhancer (black arrows) and the deletion of the intervening sequences between hs3a and hs1,2 in Δ IRIS mice totally disrupts the palindromic structure, despite the presence of all enhancer elements. Full size image The palindromic arrangement of 3’RR enhancers influences SHM Interactions with cognate antigens recruit activated B cells into germinal centres where they undergo SHM in V(D)J exons for the generation of high-affinity antibodies. SHM is strongly altered in the IgH locus of 3’RR -deficient mice, whereas SHM in light-chain loci remains unaltered [9] . We explored ΔleftPAL and Δ IRIS mice for potential SHM defects. Mice were daily immunised orally with sheep red blood cells for 2 weeks and intraperitoneally with 10 μg of LPS for 3 days. This immunisation protocol was found to be most efficient to regularly obtain in vivo -activated B cells in Peyer’s patches [8] . Mature germinal centre B cells have a B220 + Fas + GL7 + phenotype during normal immune responses to T-dependent antigens [16] . B220 + GL7 + Fas + cells were sorted from immunised wild-type ( wt ), ΔleftPAL and Δ IRIS mice. Extracted DNA was amplified by PCR and submitted to high-throughput sequencing to evaluate SHM. As SHM in light chains is not under the 3’RR control [9] , IgH SHM values along rearranged J H4 sequences were normalised to Jκ5 SHM values. Mutation frequencies of 1.45% and 0.07% were found in wt and AID −/− mice, respectively. SHM frequency was markedly reduced (by more than fourfold, at 0.33%) in ΔleftPAL mice ( Fig. 2a,b ). The presence of hs3a and hs1,2 enhancers in Δ IRIS mice maintained SHM frequency at 0.75%, that is, at an intermediate level higher than ΔleftPAL mice ( Fig. 2a,b ) but markedly lower (by about twofold) than in wt mice ( Fig. 2a,b ). Mutations were found all along the analysed 3’ J H4 DNA segment, but hotspots of mutations were evidenced in both genotypes. The proportion of transitions and transversions did not significantly differ between wt , ΔleftPAL and Δ IRIS mice ( Fig. 2c ). An increased percentage of non-mutated sequences was found in ΔleftPAL (18.9%) and Δ IRIS mice (29.1%) compared with wt mice (9.3%; Fig. 2d ). When comparing the frequency of mutations per sequence, a much lower frequency of sequences carrying multiple mutations (>10 mutations) was found in ΔleftPAL (3.1%) and Δ IRIS (1.8%) mice compared with wt mice (25.5%; Fig. 2d ). Thus, the palindromic structure of the 3’RR is instrumental for SHM of rearranged V(D)J regions, and maintaining hs3a and hs1,2 enhancers in Δ IRIS mice is not sufficient to preserve SHM at the wt level. 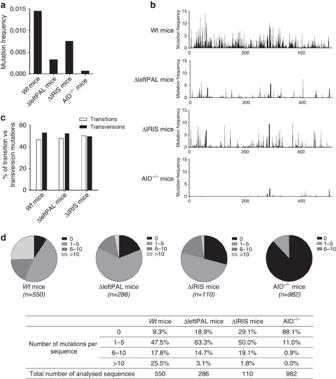Figure 2: Influence of the3’RRpalindrome on SHM. (a) SHM inVHregions of ΔleftPAL, ΔIRISandwtmice. Mice were immunised orally with sheep red blood cells for 2 weeks and intraperitoneally with 10 μg of LPS for 3 days. B220+GL7+Fas+cells from Peyer’s patches were sorted and pooled, and extracted DNA was amplified by PCR and submitted to high-throughput sequencing to evaluate SHM.VHSHM values were normalised toJκ5SHM values. Mean values from six mice for all genotypes were reported (8–12 weeks old, male and female). (b) SHM were found all along the analysed 3’JH4DNA segment and hot spot of mutations were evidenced in both genotypes. Same mice as ina. (c) The proportion of transitions and transversions did not significantly differ betweenwt, ΔleftPAL and ΔIRISmice. Same mice as ina. (d) Percentages of sequences with 0, 1–5, 6–10 and >10 mutations. (n): number of analysed sequences. Same mice as ina. Figure 2: Influence of the 3’RR palindrome on SHM. ( a ) SHM in V H regions of ΔleftPAL, Δ IRIS and wt mice. Mice were immunised orally with sheep red blood cells for 2 weeks and intraperitoneally with 10 μg of LPS for 3 days. B220 + GL7 + Fas + cells from Peyer’s patches were sorted and pooled, and extracted DNA was amplified by PCR and submitted to high-throughput sequencing to evaluate SHM. V H SHM values were normalised to Jκ5 SHM values. Mean values from six mice for all genotypes were reported (8–12 weeks old, male and female). ( b ) SHM were found all along the analysed 3’ J H4 DNA segment and hot spot of mutations were evidenced in both genotypes. Same mice as in a . ( c ) The proportion of transitions and transversions did not significantly differ between wt , ΔleftPAL and Δ IRIS mice. Same mice as in a . ( d ) Percentages of sequences with 0, 1–5, 6–10 and >10 mutations. (n): number of analysed sequences. Same mice as in a . Full size image The 3’RR palindrome influences AID recruitment We next investigated the mechanism underlying the SHM alteration. SHM correlates with transcription [17] . The partial IgH transcription defect observed in hs3b / hs4 -deficient mouse resting B cells did not lead to any significant SHM decrease in germinal centre B cells [18] . The situation is quite different in 3’RR -deficient mice, in which a partial IgH transcription defect was again observed, but then it was associated with a nearly complete V(D)J SHM blockade in activated germinal centre B cells [9] . In the present study, IgH primary transcription (location of the probe is shown in Fig. 3a ) is maintained at fairly high levels in germinal centre B cells of ΔleftPAL mice and even slightly higher in Δ IRIS mice, thus clearly uncoupling the SHM defect from any major V(D)J transcription defect ( Fig. 3b ). As positive controls, no alteration was found for Igκ transcripts (nor for AID transcripts) in ΔleftPAL and Δ IRIS mice ( Fig. 3b ). Together with transcription, modified histones, characteristic of active chromatin, constitute hallmarks of the accessibility to SHM factors. ChIP experiments (probes located are shown in Fig. 3a ) indicated that trimethylation of lysine 4 in histone H3 (H3K4me3) was markedly decreased in activated Peyer’s patch cells of ΔleftPAL mice but partially preserved in Δ IRIS mice ( Fig. 3c ). This shows a synergistic role of enhancers and of the palindromic architecture for induction of epigenetic modifications and chromatin accessibility. Stalling of RNA pol II onto the IgH V region is required for AID recruitment during SHM in germinal centre B cells. As shown in Fig. 3d , paused RNA pol II loading was markedly reduced in activated Peyer’s patch cells of ΔleftPAL mice and almost normal in Δ IRIS mice. In contrast, AID recruitment is strongly affected in both ΔleftPAL and Δ IRIS mice compared with wt mice ( Fig. 3e ). Our data thus suggest that the 3’RR palindrome strongly contributes to the efficient recruitment of AID onto the V(D)J region during SHM. 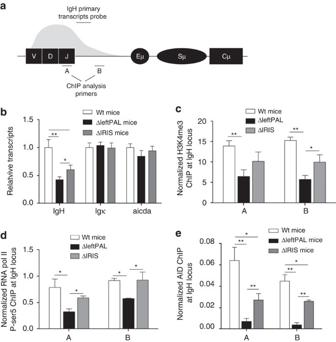Figure 3: Mechanism underlying the3’RRpalindromic effect on SHM. (a) Locations of probes (A,B) for ChIP experiments and PCR primers forIgHtranscription. (b):IgH,IgκandAICDAtranscription in ΔleftPAL, ΔIRISandwtmice. Mice were immunised orally with sheep red blood cells for 2 weeks and intraperitoneally with 10 μg of LPS for 3 days. Peyer’s patch cell RNA was extracted and transcripts were amplified by real-time PCR. Data are the mean±s.e.m. of six independent experiments with one mouse per genotype (8–12 weeks old, male and female). *P<0.05 and **P<0.001 (Mann–Whitney’sU-test for significance). Values were normalised toGAPDHtranscripts. (c) ChIP analysis of H3K4me3 inVHregions in Peyer’s patch cells in ΔleftPAL, ΔIRISandwtmice. Background ChIP signals from mock samples with irrelevant antibody were subtracted. ChIP values were normalised to the total input DNA. Data are the mean±s.e.m. of four independent experiments (8- to 12-week-old mice, male and female). *P<0.05, **P<0.01 (Mann–WhitneyU-test). ChIP experiments were done in A and B locations (as ina). Same immunisation protocol as inb. (d) ChIP analysis of pol II paused inVHregions in Peyer’s patches cells in ΔleftPAL, ΔIRISandwtmice. Data are the mean±s.e.m. of four independent experiments (8- to 12-week-old mice, male and female). *P<0.05, **P<0.01 (Mann–WhitneyU-test). Same immunisation protocol as inb. (e) ChIP analysis of AID recruitment inVHregions in Peyer’s patch cells in ΔleftPAL, ΔIRISandwtmice. Data are the mean±s.e.m. of five independent experiments (8- to 12-week-old mice, male and female). *P<0.05, **P<0.01 (Mann–WhitneyU-test). Same immunisation protocol as inb. Figure 3: Mechanism underlying the 3’RR palindromic effect on SHM. ( a ) Locations of probes (A,B) for ChIP experiments and PCR primers for IgH transcription. ( b ): IgH , Igκ and AICDA transcription in ΔleftPAL, Δ IRIS and wt mice. Mice were immunised orally with sheep red blood cells for 2 weeks and intraperitoneally with 10 μg of LPS for 3 days. Peyer’s patch cell RNA was extracted and transcripts were amplified by real-time PCR. Data are the mean±s.e.m. of six independent experiments with one mouse per genotype (8–12 weeks old, male and female). * P <0.05 and ** P <0.001 (Mann–Whitney’s U -test for significance). Values were normalised to GAPDH transcripts. ( c ) ChIP analysis of H3K4me3 in V H regions in Peyer’s patch cells in ΔleftPAL, Δ IRIS and wt mice. Background ChIP signals from mock samples with irrelevant antibody were subtracted. ChIP values were normalised to the total input DNA. Data are the mean±s.e.m. of four independent experiments (8- to 12-week-old mice, male and female). * P <0.05, ** P <0.01 (Mann–Whitney U -test). ChIP experiments were done in A and B locations (as in a ). Same immunisation protocol as in b . ( d ) ChIP analysis of pol II paused in V H regions in Peyer’s patches cells in ΔleftPAL, Δ IRIS and wt mice. Data are the mean±s.e.m. of four independent experiments (8- to 12-week-old mice, male and female). * P <0.05, ** P <0.01 (Mann–Whitney U -test). Same immunisation protocol as in b . ( e ) ChIP analysis of AID recruitment in V H regions in Peyer’s patch cells in ΔleftPAL, Δ IRIS and wt mice. Data are the mean±s.e.m. of five independent experiments (8- to 12-week-old mice, male and female). * P <0.05, ** P <0.01 (Mann–Whitney U -test). Same immunisation protocol as in b . Full size image The 3’RR palindrome weakly influences germline transcription Germline transcription (GLT) of C H gene is a known prerequisite of CSR. We evaluated GLT using real-time PCR on LPS only ( I γ3 -C γ3 , I γ2b -C γ2b ), LPS plus IL4- ( I γ1 -C γ1 ), LPS plus TGFβ- ( I α -C α ) and LPS plus INFγ- ( I γ2a -C γ2a ) activated splenic B cells from wt , ΔleftPAL and Δ IRIS mice. As shown in Fig. 4a , GLT was heterogeneously affected in ΔleftPAL mice, more or less for I γ3 -C γ3 , I γ2a -C γ2a and I γ2b -C γ2b , whereas I α -C α and I γ1 -C γ1 were preserved. Alterations were milder and restricted to I γ2a -C γ2a GLT in Δ IRIS mice ( Fig. 4a ). These data identify GLT as a basic activity of 3’RR transcriptional enhancers that can arise almost independently from their inclusion into the 3’RR palindrome. Accordingly, combined deletion of hs3b + hs4 elements, although minimally truncating the 3’RR palindrome, had a marked role in GLT [19] . It also has to be acknowledged that the various C genes are not equally affected by 3’RR defects and that C γ1 GLT was only affected by the whole 3’RR deletion [6] , [20] , whereas C α GLT is sensitive to deletions encompassing the hs4 enhancer element [6] , [21] . 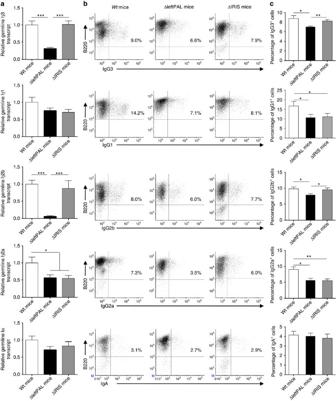Figure 4: Influence of the3’RRpalindrome on GLT and CSR. (a) GLT in B splenocytes of ΔleftPAL, ΔIRISandwtmice. Cells were stimulated with LPS±IL-4, INFγ and TGFβ for 2 days.Iγ1-Cγ1,Iγ2a-Cγ2a,Iγ2b-Cγ2b,Iγ3-Cγ3andIα-CαGL transcription was investigated by real-time PCR. Mean±s.e.m. of six independent experiments with one mouse (8–12 weeks old, male and female). *P<0.05 and ***P<0.0001 (Mann–WhitneyU-test for significance). Values were normalised toGAPDHtranscripts. (b) CSR in B splenocytes of ΔleftPAL, ΔIRISandwtmice. Cells were stimulated with LPS±IL-4, INFγ and TGFβ for 3 days. Cells were then labelled with anti-B220-APC antibodies and anti-IgG1-, anti-IgG2a-, anti-IgG2b-, anti-IgG3- and anti-IgA-FITC antibodies. One representative experiment out of six (one mouse per experiment) is shown (8- to 12-week-old mice, male and female). (c) Mean±s.e.m. of six independent experiments of CSR with one mouse (8–12 weeks old, male and female). *P<0.05 and **P<0.001 (Mann–WhitneyU-test for significance). Figure 4: Influence of the 3’RR palindrome on GLT and CSR. ( a ) GLT in B splenocytes of ΔleftPAL, Δ IRIS and wt mice. Cells were stimulated with LPS±IL-4, INFγ and TGFβ for 2 days. Iγ 1 -C γ1 , Iγ 2a -C γ2a , Iγ 2b -C γ2b , Iγ 3 -C γ3 and I α -C α GL transcription was investigated by real-time PCR. Mean±s.e.m. of six independent experiments with one mouse (8–12 weeks old, male and female). * P <0.05 and *** P <0.0001 (Mann–Whitney U -test for significance). Values were normalised to GAPDH transcripts. ( b ) CSR in B splenocytes of ΔleftPAL, Δ IRIS and wt mice. Cells were stimulated with LPS±IL-4, INFγ and TGFβ for 3 days. Cells were then labelled with anti-B220-APC antibodies and anti-IgG 1 -, anti-IgG 2a -, anti-IgG 2b -, anti-IgG 3 - and anti-IgA-FITC antibodies. One representative experiment out of six (one mouse per experiment) is shown (8- to 12-week-old mice, male and female). ( c ) Mean±s.e.m. of six independent experiments of CSR with one mouse (8–12 weeks old, male and female). * P <0.05 and ** P <0.001 (Mann–Whitney U -test for significance). Full size image The 3’RR palindrome weakly influences CSR To determine whether results on GLT translated to a decreased CSR, we appreciated by flow cytometry the number of cells switching to a particular isotype after in vitro stimulation. Flow cytometric analysis allowed the counting of cells and the study of surface expression of class-switched isotypes on LPS only, LPS plus IL4-, LPS plus TGFβ- and LPS plus INFγ-activated splenic B cells from wt and ΔleftPAL mice. A pattern almost mirroring the results of GLT (except for γ1) was found ( Fig. 4b,c ). Lowered CSR was found for IgG 3 , IgG 2a and IgG 2b , but not IgA. CSR towards IgG 1 was slightly reduced despite unchanged GLT. Maintaining the presence of all enhancer elements in Δ IRIS mice preserved CSR towards IgG 3 and IgG 2b but not IgG 2a and IgG 1 . IgA CSR was in parallel normal, similar to ΔleftPAL mice. Downstream of GLT, we observed efficient preservation of the in vitro IgG 3 and IgG 2b CSR when enhancers were maintained. Our data confirm the particular status of γ 1 and α isotypes with respect to the 3’RR -dependent regulation of CSR control. IgA CSR is only sensitive to deletion encompassing the hs4 enhancer element [6] , [20] , and recently an enhancer-RNA-expressing element called Inc-RNA-CSR was reported to promote CSR towards α by stimulating activity of the 3’RR via a long-distance interaction with the hs4 region [21] . The 3’RR palindrome and chromatin accessibility Molecular analysis of CSR has shown that the 3’RR notably promotes CSR by acting on its initial steps (GLT and histone modifications) [20] . Together with DNA transcription, several epigenetic marks involved in the targeting of the CSR machinery to S regions primed for CSR constitute hallmarks of CSR accessibility [22] , [23] . RNAseq experiments showed that C γ3 and C γ2b transcription ( Fig. 5a and d , respectively) was markedly reduced in ΔleftPAL mice compared with wt mice. The presence of hs3a and hs1,2 enhancers in Δ IRIS mice preserved C γ3 and C γ2b transcription. Levels of H3K4me3 ( Fig. 5b,e ) and H3K27ac ( Fig. 5c,f ) in the I γ3 - S γ3 - C γ3 and I γ2b -S γ2b -C γ2b regions (during IgG 3 and IgG 2b CSR, respectively) were reduced only on deletion of 3’RR enhancers but preserved in Δ IRIS mice. This suggests that 3’RR effects on CSR mostly rely on the presence of all four 3’RR enhancers, more or less independently from their rigorous palindromic arrangement. 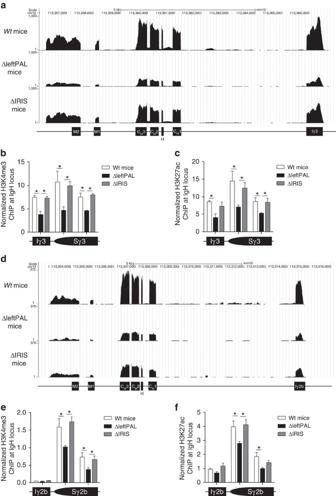Figure 5: Influence of the3’RRpalindrome onIgHtranscription and activation of epigenetic marks during CSR. (a)Iγ3-Cγ3transcription in ΔleftPAL, ΔIRISandwtmice. CD43-depleted splenocytes were cultured for 2 days with 5 μg of LPS. RNAseq experiments were performed after depletion of rRNA. Data are the mean of two independent experiments with three mice per genotype (8- to 12-week-old-male mice) (b) ChIP analysis of H3K4me3 inIγ3-Cγ3in ΔleftPAL, ΔIRISandwtmice. Data are the mean±s.e.m. of four independent experiments (8- to 12-week-old mice, male and female). *P<0.05 (Mann–WhitneyU-test). (c) ChIP analysis of H3K27ac inIγ3-Cγ3in ΔleftPAL, ΔIRISandwtmice. Data are the mean±s.e.m. of four independent experiments (8- to 12-week-old mice, male and female). *P<0.05 (Mann–WhitneyU-test). (d)Iγ2b-Cγ2btranscription (RNAseq experiments) in ΔleftPAL, ΔIRISandwtmice. Same mice as ina. (e) ChIP analysis of H3K4me3 inIγ2b-Cγ2bin ΔleftPAL, ΔIRISandwtmice. Data are the mean±s.e.m. of four independent experiments (8- to 12-week-old mice, male and female). *P<0.05 (Mann–WhitneyU-test). (f) ChIP analysis of H3K27ac inIγ2b-Cγ2bin ΔleftPAL, ΔIRISandwtmice. Data are the mean±s.e.m. of four independent experiments (8- to 12-week-old mice, male and female). *P<0.05 (Mann–WhitneyU-test). Figure 5: Influence of the 3’RR palindrome on IgH transcription and activation of epigenetic marks during CSR. ( a ) Iγ 3 -C γ3 transcription in ΔleftPAL, Δ IRIS and wt mice. CD43-depleted splenocytes were cultured for 2 days with 5 μg of LPS. RNAseq experiments were performed after depletion of rRNA. Data are the mean of two independent experiments with three mice per genotype (8- to 12-week-old-male mice) ( b ) ChIP analysis of H3K4me3 in I γ 3 -C γ3 in ΔleftPAL, Δ IRIS and wt mice. Data are the mean±s.e.m. of four independent experiments (8- to 12-week-old mice, male and female). * P <0.05 (Mann–Whitney U -test). ( c ) ChIP analysis of H3K27ac in Iγ 3 -C γ3 in ΔleftPAL, Δ IRIS and wt mice. Data are the mean±s.e.m. of four independent experiments (8- to 12-week-old mice, male and female). * P <0.05 (Mann–Whitney U -test). ( d ) Iγ 2b -C γ2b transcription (RNAseq experiments) in ΔleftPAL, Δ IRIS and wt mice. Same mice as in a . ( e ) ChIP analysis of H3K4me3 in Iγ 2b -C γ2b in ΔleftPAL, Δ IRIS and wt mice. Data are the mean±s.e.m. of four independent experiments (8- to 12-week-old mice, male and female). * P <0.05 (Mann–Whitney U -test). ( f ) ChIP analysis of H3K27ac in Iγ 2b -C γ2b in ΔleftPAL, Δ IRIS and wt mice. Data are the mean±s.e.m. of four independent experiments (8- to 12-week-old mice, male and female). * P <0.05 (Mann–Whitney U -test). Full size image The 3’RR palindrome and B-cell fate The full deletion of the 3’RR was reported to affect membrane IgM density and to modulate the B-cell fate towards less marginal zone B cells [5] . We generated heterozygous IgH a ΔleftPAL /b wt mice and IgH a Δ IRIS /b wt mice by crossing homozygous ΔleftPAL mice ( IgH a ΔleftPAL /a ΔleftPAL ) and ΔIRIS mice ( IgH a Δ IRIS /a Δ IRIS ) with C57BL/6 mice ( IgH b wt /b wt ). Analysis of splenic B cells with IgM-allotype-specific antibodies indicated similar percentages of transitional B cells (B220 + AA4.1 + ), follicular B cells (B220 + CD21 low CD23 high ) and marginal zone B cells (B220 + CD21 high CD23 low ) expressing either the a or b allotype in a ΔleftPAL /b wt and IgH a Δ IRIS /b wt mice ( Fig. 6a,b ) and no defect in membrane IgM density ( Fig. 6c ). Percentages of B220 + CD138 + plasmablasts were not different in ΔleftPAL, Δ IRIS and wt mice ( Fig. 6d ). The lowered IgM density observed in CD138 + plasmablasts is almost restored in Δ IRIS mice ( Fig. 6e ). This again suggests that most of the effects of 3’RR enhancers on IgM expression and relevant B-cell fate are simply provided by the presence of all four 3’RR enhancers, without requiring their rigorous palindrome arrangement. 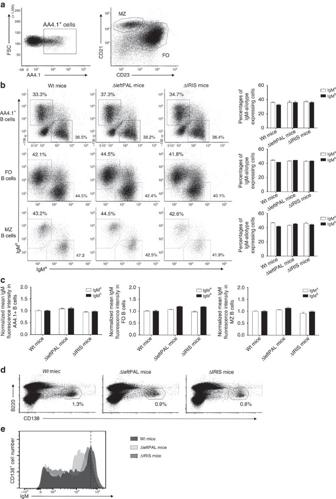Figure 6: Influence of the3’RRpalindrome on BCR expression and B-cell fate. (a) Flow cytometry analysis of transitional (TR) B cells (AA4.1+), follicular (FO) B cells (CD21lowCD23high) and marginal zone (MZ) B cells (CD21highCD23low). One representative experiment out of five is shown (8- to 12-week-old mice, male and female). (b) TR, FO and MZ B cells expressing theaorballele in aΔleftPAL/bwt, aΔIRIS/bwtand awt/bwtmice. One representative experiment out of five is shown (left part). Mean±s.e.m. of five mice for all genotypes (right part; 8–12-week-old mice, male and female). (c) Mean±s.e.m. of membrane IgM densities on TR, FO and MZ B cells expressing theaorballele in aΔleftPAL/bwt, aΔIRIS/bwtand awt/bwtmice (8–12-week-old mice, male and female). (d) Flow cytometry analysis of plasmablasts (B220+CD138+) in spleen of homozygous aΔleftPAL/bwt, aΔIRIS/bwtand awt/bwtmice. One representative experiment out of three is shown (8- to 12-week-old mice, male and female). (e) Expression of IgM on plasmablasts of homozygous ΔleftPAL, ΔIRIS andwtmice. One representative experiment out of three is shown (8- to 12-week-old mice, male and female). Figure 6: Influence of the 3’RR palindrome on BCR expression and B-cell fate. ( a ) Flow cytometry analysis of transitional (TR) B cells (AA4.1 + ), follicular (FO) B cells (CD21 low CD23 high ) and marginal zone (MZ) B cells (CD21 high CD23 low ). One representative experiment out of five is shown (8- to 12-week-old mice, male and female). ( b ) TR, FO and MZ B cells expressing the a or b allele in a ΔleftPAL /b wt , a ΔIRIS /b wt and a wt /b wt mice. One representative experiment out of five is shown (left part). Mean±s.e.m. of five mice for all genotypes (right part; 8–12-week-old mice, male and female). ( c ) Mean±s.e.m. of membrane IgM densities on TR, FO and MZ B cells expressing the a or b allele in a ΔleftPAL /b wt , a ΔIRIS /b wt and a wt /b wt mice (8–12-week-old mice, male and female). ( d ) Flow cytometry analysis of plasmablasts (B220 + CD138 + ) in spleen of homozygous a ΔleftPAL /b wt , a ΔIRIS /b wt and a wt /b wt mice. One representative experiment out of three is shown (8- to 12-week-old mice, male and female). ( e ) Expression of IgM on plasmablasts of homozygous ΔleftPAL, ΔIRIS and wt mice. One representative experiment out of three is shown (8- to 12-week-old mice, male and female). Full size image The 3’RR palindrome and Ig synthesis Ig production was assessed in vitro through stimulation of splenocytes with LPS and/or cytokines. It was significantly affected in both mutant strains of mice, although this phenotype was aggravated in ΔleftPAL mice lacking two enhancers. IgG 2b (LPS stimulation), IgG 1 (LPS+IL4 stimulation), IgG 2a (LPS+INFγ stimulation) and IgA (LPS+TGFβ stimulation) syntheses were markedly reduced in ΔleftPAL compared with wt mice ( Fig. 7a ). Similar alterations were observed in Δ IRIS mice, except that they were eventually less pronounced and spared IgG 3 and IgA secretion ( Fig. 7a ). We next investigated Ig production and plasma accumulation in vivo and again found similar alterations in both mutant strains, which mostly showed defects for IgM, IgG 3 and IgG 2a plasma levels, whereas IgG 1 , IgG 2b and IgA were preserved ( Fig. 7b ). Although statistically significant in both cases, the plasma IgG 3 and IgG 2a levels were less markedly decreased in Δ IRIS mice than in mice with the dual deletion of hs3b and hs4 enhancers [19] . Although these total Ig-level defects were clear, evaluation of specific circulating antibody levels after ovalbumin immunisation did not show major alteration, neither in ΔleftPAL nor in Δ IRIS mice, suggesting that the intrinsic B-cell defect was compensated on specific antigenic challenge (with potentially a trend of lower levels of IgG1 and IgG2a antibodies in mutant animals; Fig. 7c ). 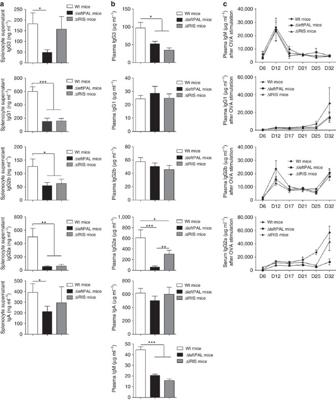Figure 7: Influence of the3’RRpalindrome on Ig synthesis. (a) ELISA analysis of IgG1, IgG2a, IgG2b, IgG3and IgA in supernatants of LPS±IL-4-, INFγ- and TGFβ-stimulated splenocytes of ΔleftPAL, ΔIRISandwtmice. Data are the mean±s.e.m. of eight experiments with one mouse (8–12 weeks old, male and female). *P<0.05, **P<0.01 and **P<0.001 (Mann–WhitneyU-test for significance). (b) ELISA analysis of IgM, IgG1, IgG2a, IgG2b, IgG3and IgA in plasma of 10 ΔleftPAL, 9 ΔIRISmice and 18wtmice (8 weeks old, male and female). Mean±s.e.m. *P<0.05, **P<0.01 and **P<0.001 (Mann–WhitneyU-test for significance). (c) Ovalbumin-specific IgM, IgG1, IgG2aand IgG2b. Antibody levels, detected by ELISA, are expressed in arbitrary units by comparison with control plasma values. Time after immunisation is indicated in days. Each point is the mean±s.e.m. of plasma determinations from six mice for each genotype (8–12 weeks old, male and female). One representative experiment out of two is shown. Figure 7: Influence of the 3’RR palindrome on Ig synthesis. ( a ) ELISA analysis of IgG 1 , IgG 2a , IgG 2b , IgG 3 and IgA in supernatants of LPS±IL-4-, INFγ- and TGFβ-stimulated splenocytes of ΔleftPAL, Δ IRIS and wt mice. Data are the mean±s.e.m. of eight experiments with one mouse (8–12 weeks old, male and female). * P <0.05, ** P <0.01 and ** P <0.001 (Mann–Whitney U -test for significance). ( b ) ELISA analysis of IgM, IgG 1 , IgG 2a , IgG 2b , IgG 3 and IgA in plasma of 10 ΔleftPAL, 9 Δ IRIS mice and 18 wt mice (8 weeks old, male and female). Mean±s.e.m. * P <0.05, ** P <0.01 and ** P <0.001 (Mann–Whitney U -test for significance). ( c ) Ovalbumin-specific IgM, IgG 1 , IgG 2a and IgG 2b . Antibody levels, detected by ELISA, are expressed in arbitrary units by comparison with control plasma values. Time after immunisation is indicated in days. Each point is the mean±s.e.m. of plasma determinations from six mice for each genotype (8–12 weeks old, male and female). One representative experiment out of two is shown. Full size image The IgH 3’RR is a large and complex cis -regulatory region with a unique and striking palindromic architecture ( Fig. 1 ) for which a potential functional role has been long questioned. Because the previously reported focal genomic alterations of the 3’RR could not address the issue of a role for the 3’RR architecture [6] , [19] , [24] , [25] , [26] , [27] ( Fig. 8 ), we generated two different mice with complete disruption of the palindromic architecture, either by globally deleting the first-half part of the 3’RR (including hs3a and hs1,2 enhancers) or by removing all inverted repeats while preserving all enhancers (but with hs3 enhancer disposed as direct repeats) and compared them. SHM in V H genes was markedly affected by the palindromic deconstruction. Keeping hs3a and hs1,2 enhancer intact in Δ IRIS mice prevented the fall in histone modification and RNA pol II pausing but nevertheless affected AID recruitment in V H genes. Taken together, this indicates that, even when all enhancer elements were present, breaking the palindrome symmetry by deleting half of inter-enhancer intervening sequences plus flipping hs3a in a direct repeat orientation affected SHM at a level similar to ΔleftPAL mice also lacking hs3a and hs1,2 . Although a role for the non-conserved intervening sequences by themselves cannot be excluded, these data strongly suggest a role for the palindromic 3’RR architecture during SHM. Indeed, although the absence of any inter-species sequence identity between 3’RR IRIS suggests that they do not include major functional motif, conservation of their dyad symmetry architecture around hs1,2 by contrast suggests an evolutionary pressure on the palindromic structure itself [15] . Our data fully support the idea that this pressure on the 3’RR architecture connects with a functional importance for germinal centre B-cell response and thus for optimal humoral immunity. On the basis of previously published data, one can also suggest that the IgH 3’RR is somehow split into functional modules. The 25-kb-long palindrome seems to have a strong role in SHM, whereas hs4 deletion alone only affected membrane IgM expression in resting B cells [27] , and the hs3b + hs4 deletion affected IgM expression and CSR but not SHM [18] , [19] . These data do not formally exclude the hypothesis that the reduction in distances between the enhancers alone accounts for our SHM observation. For other enhancers, dependence on proper spatial organisation and spacing has been reported [28] . However, we think that data regarding the 3’RR are much more in favour of an architectural role of the repeats, contributing to a given functional secondary or tertiary structure of either the 3’RR and/or the whole IgH locus. A contribution of transcription to 3’RR conformation is also suggested by our previous characterisation of 3’RR eRNA [8] , and the recent demonstration that long non-coding RNA coming from distal IncRNA-CSR element positively regulates the activity of the 3’RR (ref. 21 ). 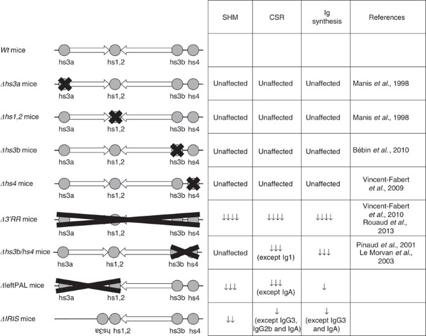Figure 8: Mutants of the3’RRenhancers. References and main results are reported and compared with ΔleftPAL and ΔIRISmice. Figure 8: Mutants of the 3’RR enhancers. References and main results are reported and compared with ΔleftPAL and Δ IRIS mice. Full size image Combined effect of the four 3’RR enhancers was not sufficient alone for an efficient AID recruitment and thus for a normal SHM rate. Interestingly, a previously reported 3'RR deletion sparing most of its palindromic part but removing its two last enhancers ( hs3b + hs4 ) had no effect on SHM [18] , but it had major effects on CSR [9] , whereas complete deletion of the 3’RR was shown to simultaneously affect CSR and SHM [6] , [9] . In the present study, analysis of ΔleftPAL and Δ IRIS mice with a deconstruction of the 3’RR palindrome only had a minor effect on CSR with reduced CSR towards γ 3 and γ 2b connected with decreased γ 3 and γ 2b GLT. The 3’RR -induced CSR control is complex, as CSR towards α is mostly dependent on the hs4 enhancer [21] , and as CSR to γ 1 appears as at least partially 3’RR -independent [6] , [20] . These differences probably relate to the specific structures of germline promoters and of S regions, as the number of G-clusters to initiate R loops, the number of WGCW sites for AID deamination and distance to promoter are of key importance for CSR efficiency [29] . Thereby, S α has been demonstrated to be able to form R-loops more readily than other isotypes, thus allowing AID to induce the double-strand breaks (DSBs) required to initiate CSR, because of the short distance between I α and C α (ref. 30 ). Transcription is suggested to play a key role both in SHM and CSR. However, the induction of these two processes is different. Although CSR relies mostly on transcription and the repetitive sequences of S regions to produce ssDNA and recruit AID, SHM requires the presence of many co-factors for efficient AID targeting and, thus, may be more dependent on the 3D structure of the 3’RR , which may allow a precise regulation of this mechanism. Moreover, CSR is a ‘yes’ or ‘no’ process, which might still be able to occur even when the frequency of AID lesions within downstream S region is decreased (especially in conditions with a 3’RR deletion, where double-strand breaks still occur at high rate in the upstream S μ region [20] . In addition, CSR and SHM require the activity of different parts of the AID molecule and different partners of AID, such as 14-3-3 and KAP1/HP1 in the case of CSR [31] . Finally, it has been demonstrated that V and S regions use different mechanisms to expose ssDNA to AID. Although S regions form long R-loops because of to the high level of transcription and their repetitive sequence, V regions display short patches of ssDNA that require the assembly of protein–DNA complex [32] . AID is, evolutionarily, the first enzyme known to improve immune diversity by SHM, and it is present as early as the primordial jawed vertebrates; AID-induced CSR begins later, with the first amphibians [32] , [33] , [34] . In conclusion, SHM requires both 3’RR enhancers and its palindromic architecture, whereas CSR relies mostly on the enhancers, which are sufficient for GLT and accessibility of the locus. Inverted repeats may function by positioning the 3’RR in its optimal 3D configuration, together with eRNA, IncRNA and transcription factor in order to stabilise the chromosomal loops that most efficiently recruit AID downstream of pV H promoters [35] . It is of interest to note that CSR and the increased IgH transcription occurring at the plasma cell stages do not require these elements, reinforcing the concept that CSR and SHM are mechanistically differently controlled by the 3’RR . Understanding differences of the pathways that contribute to CSR and SHM will help us understand the mechanisms for antibody regulation and diversity. Our present results indicate that the 3’RR regulates AID-induced SHM and CSR by different mechanisms, underline the complexity of action of this major cis -regulatory element and demonstrate that not only enhancers included in the 3’RR but also the global palindromic architecture of this region are critical determinants of its function. Mice In all, 129 wt mice and C57Bl/6 wt mice (from Charles Rivers Laboratories, France), as well as ΔLeftPAL and Δ IRIS mice (from UMR CNRS 7276, Limoges, France; in a 129 background), were used. Our research has been approved by our local ethics committee review board (Comité Régional d'Ethique sur l'Expérimentation Animale du Limousin, Limoges, France) and has been carried out according to the European guidelines for animal experimentation. Vector construction and embryonic stem cell screening A neomycin-resistance gene ( neo R ) flanked by loxP sites was stuck in between 5’ and 3’ arms. At the 5’ end, a phosphoglucokinase promoter-herpes simplex virus thymidine kinase gene ( Tk ) was included to permit negative selection against random integration. Cells of the embryonic stem (ES) cell line E14 were transfected with linearised vector by electroporation and selected using 300 μg ml −1 geneticin and 2 μg ml −1 gancyclovir. The ES cell line E14 was derived from the inbred mouse strain 129. PCR analysis with primers 5’ and 3’ of the construct identified recombinants. ES clones showing homologous recombination were injected into C57Bl/6 blastocysts, and the resulting chimeras were mated with C57Bl/6 animals. Germline transmission in heterozygous mutant mice was checked by specific PCR. Mutant mice were mated with cre-transgenic mice. The progeny was checked by PCR for the occurrence of a cre-mediated deletion of the neo R gene. ΔleftPAL and Δ IRIS homozygous mice were checked by PCR. The various PCR primers used for screening the ΔleftPAL and Δ IRIS mice are reported in the Supplementary Table 1 and located in the Supplementary Fig. 1 . Blood sampling Blood samples were recovered from transgenic mice and wt controls with heparinised needles. Ten-week-old animals (male and female) were used. Plasma samples were recovered by centrifugation and stored at −20 °C until use. Spleen cell cultures for CSR and Ig determinations Single-cell suspensions of CD43 − spleen cells of wt , ΔleftPAL and Δ IRIS mice (8–12 weeks old, male and female) were cultured for 3 days at 1 × 10 6 cells per ml in RPMI 1640 with 10% fetal calf serum, 5 μg ml −1 LPS with or without 20 ng ml −1 IL-4, 2 ng ml −1 TGFβ and 2 ng ml −1 INFγ (PeproTech, Rocky Hill, NJ) [6] , [36] . At day 3, 1 × 10 6 cells were cultured for 24 h in growth medium without LPS+cytokine. Supernatants were recovered and stored at −20 °C until use. At day 3, cultured splenic B cells were incubated with anti-B220-SpectralRed (PC5)-labelled antibodies (Biolegend, ref: 103212) and anti-IgG 1 - (ref: 107020), anti-IgG 2a - (ref: 108002), anti-IgG 2b - (ref: 109002), anti-IgG 3 - (ref: 110002) and anti-IgA- (ref: 104002) fluorescein-isothiocyanate (FITC)-labelled antibodies (Southern Biotechnologies), and then analysed on a Fortessa LSR2 (Beckton-Dickinson) [6] . All antibodies were at a concentration of 10 μg ml −1 . Real-time quantitative PCR of I x -C x GL transcription Three-day in vitro -stimulated splenocytes (LPS+appropriated cytokines) were collected and RNA was extracted for investigation of I x -C x transcripts. RNA and cDNA were prepared using standard techniques. Quantitative PCR was performed using power SYBR green (Applied Biosystems). PCR primers used for determinations of I x -C x transcripts are reported in the Supplementary Table 1 . Immunisation For immunisation experiments, batches of 8-week-old mice were used (6 mice per genotype, male and female). The first immunisation was performed with 50 μg of chicken ovalbumin per animal in 50% complete Freund’s adjuvant and a second immunisation was performed 13 days later with the same amount of antigen in 50% incomplete Freund adjuvant. Immunised mice were eye-bled at various intervals during the immunisation protocol, and plasma was analysed for the presence of ovalbumin-specific IgM, IgG 1 , IgG 2a and IgG 2b by ELISA [18] . Antibody determinations Specific ELISAs were performed as follows [6] , [18] : ELISAs for specific IgM, IgG 1 , IgG 2a and IgG 2b were performed in polycarbonate 96-multiwell plates coated overnight at 4 °C with 100 μl of 10 mg ml −1 ovalbumin solution in 0.05 M Na 2 CO 3 buffer. After washing, a blocking step was performed with gelatin (2 mg ml −1 ) in PBS buffer. After washing, 50 μl of assayed plasma or control plasma was diluted into successive wells (first dilution to 1:50) in gelatin (2 mg ml −1 ) in PBS buffer and incubated for 2 h at 37 °C. The positive control consisted of a pool of plasma from ovalbumin-immunised wt mice (the same control plasma was used in all ELISAs). After washing, 100 μl per well of appropriate conjugated antibodies were added and adsorbed for 2 h at 37 °C. Alkaline phosphatase (AP)-conjugated goat antisera specific for mouse IgM (Southern Biotechnologies, ref: 102104), IgG 1 (Southern Biotechnologies, ref: 107004), IgG 2a (Southern Biotechnologies, ref: 1080004) and IgG 2b (Beckman Coulter, ref: 731943) were used at a concentration of 1 μg ml −1 . After washing, AP activity was assayed using AP substrate, and enzymatic reactions were stopped with 3 M NaOH. The optical density was measured at 400 nm. Diluted plasmas were compared with the titration curve obtained on the same multiwell plate, which allowed the quantification of ovalbumin-specific antibodies in arbitrary units. Culture supernatants and plasma (first dilution to 1:50) from ΔleftPAL, Δ IRIS and wt mice were analysed for the presence of the various Ig classes (IgM, IgG 1 , IgG 2b , IgG 2b , IgG 3 and IgA) by ELISA, as previously described above [6] , [18] , [20] , except for the coating made with suitable capture antibodies (2 μg ml −1 for IgM (Southern Biotechnologies, ref: 902001), IgG 1 (Southern Biotechnologies, ref: 107001), IgG 2a (Southern Biotechnologies, ref: 731956) and IgG 2b (Southern Biotechnologies, ref: 731940), 3 μg ml −1 for IgG 3 (Southern Biotechnologies, ref: 732371) and 4 μg ml −1 for IgA (Southern Biotechnologies, ref: 104001), blocking performed with 3% BSA in PBS, AP-conjugated goat antisera specific for mouse IgA (Southern Biotechnologies, ref: 104004) and IgG 3 (Beckman Coulter, ref: 732374), and for standards made with specific antisera for IgM, IgG 1 , IgG 2a , IgG 2b , IgG 3 and IgA (Southern Biotechnologies)). ChIP experiments Mice immunisations were performed orally with sheep red blood cells for 2 weeks and intraperitoneally with 10 μg of LPS for 1 week (8–12 weeks old, male and female). ChIP experiments were done on freshly isolated Peyer’s patches cells, as previously described [8] . In brief, 4 × 10 6 B cells were cross-linked at room temperature for 15 min in 15 ml of PBS with 1% formaldehyde. The reaction was quenched with 0.125 M glycine. After lysis, chromatin was sonicated to 0.5–1 kb using a Vibracell 75043 (Thermo Fisher Scientific). After dilution in ChIP buffer (0.01% SDS, 1.1% Triton X-100, 1.2 mM EDTA, 16.7 mM Tris-HCl, pH 8.1 and 167 mM NaCl), chromatin was precleared by rotating for 2 h at 4 °C with 50 ml of 50% protein A/G slurry (0.2 m ml −1 sheared salmon sperm DNA, 0.5 m ml −1 BSA and 50% protein A/G; Sigma). In all, 0.1 × 10 6 cell equivalents were saved as input, and 2 × 10 6 cell equivalents were incubated overnight with anti-AID or control antibodies. Immune complexes were precipitated by the addition of protein A/G. Cross-linking was reversed by overnight incubation (70 °C) in TE buffer with 0.02% SDS, and chromatin was phenol/chloroform extracted. Anti-AID antibodies were kindly provided by Dr P. Gearhart. Anti-H3K4me3 was obtained from Millipore (ref: 07473), and anti-K3K27ac and anti-P-ser5 pol II pause were obtained from Abcam (clone ab4729 and ab5131, respectively). PCR primers are detailed in Supplementary Table 1 . IgH primary transcription analysis Total RNA was phenol–chloroform-extracted from 5 × 10 5 B cells from freshly isolated peyers patches, in mice previously stimulated, as described above for SHM analysis. Real-time PCR was performed in duplicate by using TaqMan assay reagents and analysed on a StepOnePlus RT PCR system (Applied Biosystems). IgH primary transcripts (probe located in the intron between the last J H and the intronic Eμ enhancer) were studied as previously reported [37] . Forward primer, 5′-TTCTGAGCATTGCAGACTAATCTTG-3′; reverse primer, 5′-CCTAGACAGTTTATTTCCCAACTTCTC-3′; and probe, 5′-CCCTGAGGGAGCCG-3′. κ-primary transcripts (probe located in the intron between the last Jκ and the intronic enhancer Ei κ): κ-forward primer, 5′-ACCCCCGCGGTAGCA-3′; κ-reverse primer, 5′-TCCTATCACTGTGCCTCAGGAA-3′; and probe, 5′-CCCTTGCTCCGCGTGGACCA-3′. Aicda transcripts were also analysed (reference Mm01184115-m1) and GAPDH was used for the normalisation of gene expression levels (reference Mm99999915-g1). Sequencing Mice were immunised orally with sheep red blood cells for 2 weeks and intraperitoneally with 10 μg of LPS for 3 days. Single-cell suspensions from Peyer’s patches were labelled with B220-APC- (Biolegend, ref:103212), GL7-FITC- (Beckton Dikinson, ref: 561530) and Fas-PE- (Beckton Dikinson, ref: 554258) conjugated antibodies. Purification of B220 + GL7 + Fas + cells was realized on a FACS ARIA III (BD). Genomic DNA was extracted, and a region corresponding to a sequence of 517 bp downstream of the J H4 segment was amplified by PCR. As a control, Igκ light-chain VJ -rearranged fragments were also amplified. Primers (detailed in the Supplementary Table 1 ) were coupled to 454 Sequencing adaptor sequences and PCR was performed using the program previously reported [8] . According to the manufacturer, the resulting purified amplicons were prepared for sequencing with a GS Junior Titanium emPCR Kit (Lib-A; Roche), and the library of DNA fragments was sequenced on a 454 GS Junior instrument (Roche). Obtained sequences were aligned to the reference sequence using BWA aligner [38] , and SAMtools software was used to obtain BAM files [39] . Redundant sequences were excluded, and wig files were generated using IGV Tools [40] and manually analysed to determine mutation frequencies for each nucleotide in the sequence. RNAseq experiments CD43 − splenocytes were obtained from 4 wt , 4 ΔleftPAL and 4 Δ IRIS mice before and after 48 h of in vitro stimulation (1 × 10 6 cells per ml in RPMI 1640 with 10% fetal calf serum) with 5μg ml −1 LPS. RNA was extracted using the miRNeasy kit from QIAGEN, according to the manufacturer’s instructions. Two pooled RNAs (with two samples) were obtained for each genotype. RNA libraries were obtained using TruSeq Stranded Total RNA with Ribo-Zero Gold (Illumina), according to the manufacturer’s instruction. Libraries were sequenced on a NextSeq500 sequencer, using NextSeq 500/550 High Output Kit (Illumina). Illumina NextSeq500 paired-end 2 × 150-nt reads were mapped with STAR release v2.4.0a versus mm10 with gene model from Ensembl release 77 with default parameters. Quantification of genes was then performed using feature Counts release subread-1.4.6-p1-Linux-x86_64 with ‘--primary -g gene_name -p -s 1 -M ’ options based on Ensembl GTF release 77 annotations. Accession codes: The RNA-seq data derived from the CD43 − splenocytes has been deposited at the GEO under the accession code GSE76359 . How to cite this article: Saintamand, A. et al . Deciphering the importance of the palindromic architecture of the immunoglobulin heavy chain 3’ regulatory region. Nat. Commun. 7:10730 doi: 10.1038/ncomms10730 (2016).